Electrically tuned magnetic order and magnetoresistance in a topological insulator The interplay between topological protection and broken time reversal symmetry in topological insulators may lead to highly unconventional magnetoresistance behaviour that can find unique applications in magnetic sensing and data storage. However, the magnetoresistance of topological insulators with spontaneously broken time reversal symmetry is still poorly understood. In this work, we investigate the transport properties of a ferromagnetic topological insulator thin film fabricated into a field effect transistor device. We observe a complex evolution of gate-tuned magnetoresistance, which is positive when the Fermi level lies close to the Dirac point but becomes negative at higher energies. This trend is opposite to that expected from the Berry phase picture, but is intimately correlated with the gate-tuned magnetic order. The underlying physics is the competition between the topology-induced weak antilocalization and magnetism-induced negative magnetoresistance. The simultaneous electrical control of magnetic order and magnetoresistance facilitates future topological insulator based spintronic devices. The studies of magnetoresistance (MR) in novel magnetic materials have been at the center stage in the field of spintronics [1] . The most notable example is the discovery of giant MR when two ferromagnetic (FM) films separated by a nonmagnetic spacer layer have anti-parallel alignment [2] . Giant MR not only reveals the remarkable consequence of spin-dependent transport, but also caused a revolution in information technology. The recently discovered topological insulators (TIs) possess Dirac-like surface states that are protected by time reversal symmetry (TRS) and exhibit a host of novel properties [3] , [4] , [5] . Introducing magnetism into TI, which breaks the TRS, is expected to create exotic topological magnetoelectric effects [6] , [7] , [8] , [9] , [10] . In a naïve picture, a TI film with long-range FM order can be viewed as a bulk ferromagnet sandwiched between two layers of Dirac fermions with opposite chiralities, as illustrated in Fig. 1a . The MR behaviour in such a system is apparently of tremendous interest, but experimental challenges associated with magnetically doped TI have hindered a thorough exploration of this phenomenon. For example, recent studies show that Cr-doped Bi 2 Se 3 , which is presumably the best TI, remains paramagnetic in spite of increased Cr content [11] . Transition metal-doped Sb 2 Te 3 exhibit robust FM order [12] , [13] , but the charge transport is dominated by bulk carriers rather than the topological surface states. The most ideal situation, of course, is to have a TI film with spontaneous FM order and tunable Fermi level ( E F ) over a wide doping range across the Dirac Point (DP). 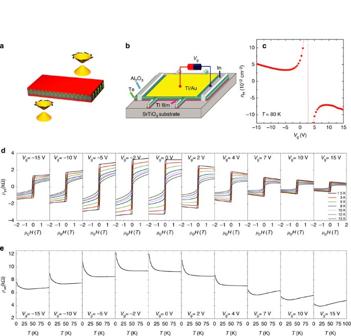Figure 1: Measurement setup and electrical characterization of the field effect transistor. (a) A FM TI thin film consists of two layers of Dirac fermions separated by the bulk FM layer. The Dirac fermions residing on the two surfaces have opposite spin chirality. A gap is opened at the DP due to the out-of-plane ferromagnetism. (b) Schematic device for the magnetotransport measurement of the Cr0.15(Bi0.1Sb0.9)1.85Te3thin film. A Hall bar geometry is used to measure theρxxandρyxsimultaneously under various gate voltages and magnetic field. (c) Electric field dependence of carrier density at 80 K. Carrier density is estimated from the Hall curve at 80 K. The carrier density shows divergent behaviour aroundVg=+2 V. (d) Temperature dependence of the anomalous Hall effect under various gate voltages. Strong FM order is confirmed by the square-shaped hysteresis at 1.5 K over all the gate voltages. The ordinary Hall slope evolves from positive to the negative when theEFis tuned across the DP. (e) Temperature dependence of 2D longitudinal resistivity under varied gate voltages. The highTmetallic behaviour at large |Vg| gradually becomes insulating asEFis tuned into the bulk gap by the gate voltage. Figure 1: Measurement setup and electrical characterization of the field effect transistor. ( a ) A FM TI thin film consists of two layers of Dirac fermions separated by the bulk FM layer. The Dirac fermions residing on the two surfaces have opposite spin chirality. A gap is opened at the DP due to the out-of-plane ferromagnetism. ( b ) Schematic device for the magnetotransport measurement of the Cr 0.15 (Bi 0.1 Sb 0.9 ) 1.85 Te 3 thin film. A Hall bar geometry is used to measure the ρ xx and ρ yx simultaneously under various gate voltages and magnetic field. ( c ) Electric field dependence of carrier density at 80 K. Carrier density is estimated from the Hall curve at 80 K. The carrier density shows divergent behaviour around V g =+2 V. ( d ) Temperature dependence of the anomalous Hall effect under various gate voltages. Strong FM order is confirmed by the square-shaped hysteresis at 1.5 K over all the gate voltages. The ordinary Hall slope evolves from positive to the negative when the E F is tuned across the DP. ( e ) Temperature dependence of 2D longitudinal resistivity under varied gate voltages. The high T metallic behaviour at large | V g | gradually becomes insulating as E F is tuned into the bulk gap by the gate voltage. Full size image In this work, we achieve these goals by growing magnetically doped TI film with chemical formula Cr 0.15 (Bi 0.1 Sb 0.9 ) 1.85 Te 3 and fabricating it into a field effect transistor device, as schematically drawn in Fig. 1b . The mixing of Bi/Sb can tune the band structure close to an ideal TI [14] , and when doped with Cr, the system exhibits bulk FM order with out-of-plane easy axis [15] . The electrical gate can drive E F to various regimes of the TI band structure. Details about sample growth, device fabrication and measurements are presented in Methods and Supplementary Note 1 . Our transport measurements on such a field effect transistor device reveal an unusually complex evolution of MR when E F is tuned across the DP by gate voltage. In particular, MR tends to be positive when E F lies close to the DP but becomes negative at higher energies. This trend is opposite to that expected from the Berry phase picture for localization, but is intimately correlated with the gate-tuned magnetic order. We show that the underlying physics is the competition between the topology-induced weak antilocalization (WAL) and magnetism-induced negative MR. The simultaneous electrical control of magnetic order and magnetotransport facilitates future TI-based spintronic devices. Demonstration of FM order in the sample Figure 1d displays the temperature ( T ) dependent two-dimensional (2D) Hall resistivity ( ρ yx ) measured at varied gate voltages ( V g ). At the lowest T =1.5 K, the square-shaped hysteretic Hall traces for all V g indicate robust FM order. The total ρ yx in this case can be expressed as ρ yx = R A M + R H H . Here, M is the magnetization of the sample and R A / R H is the anomalous/ordinary Hall coefficient, respectively. With increasing V g from −15 V to +15 V, the R H at T =1.5 K changes from positive to negative, indicating the change from p- to n -type charge carriers via the bulk insulating regime. The existence of robust ferromagnetism across the entire V g range is similar to that observed in Cr-doped (Bi,Sb) 2 Te 3 films with varied Bi/Sb ratio [15] . The FM order becomes weaker with increasing T and disappears for all V g at T =15 K, when the Hall curves become reversible but retain strong nonlinearity due to strong FM fluctuations. The gate tuning of carrier density can be best demonstrated by the Hall measurements at T =80 K (See Supplementary Note 1 for details), when the influence of FM fluctuation is much reduced. Figure 1c shows the V g -dependent nominal carrier density n H estimated from the ordinary Hall coefficient R H as n H =1/ R H . The most dramatic feature here is the divergent behaviour around V g =+2 V, when the sample is in the charge neutral regime with E F lying close to the DP [16] . On the left (right) side, E F lies below (above) the DP with hole-type (electron-type) carriers tuned systematically by V g . At the large V g limit close to ±15 V, the bulk band carriers start to dominate the charge transport. The same trend is revealed by the longitudinal resistivity ρ xx measured under varied gate voltages. As shown in Fig. 1e , at V g =±15 V, the ρ xx shows a metallic behaviour at high T and becomes weakly insulating at low T . As E F is tuned towards the DP, the ρ xx value keeps rising and the high T behaviour gradually becomes insulating between V g =−2 V and +4 V. These results are consistent with the Hall effect measurements and confirm that the bulk is insulating in this regime but becomes metallic at higher V g . 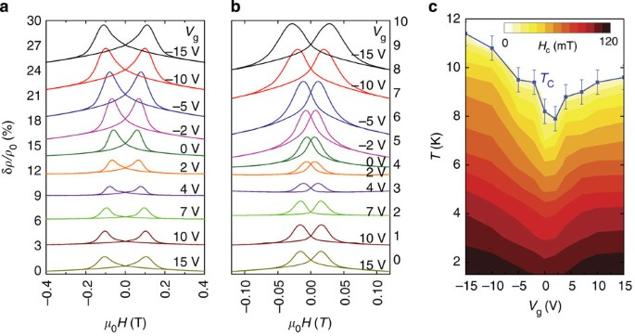Figure 2: Magnetotransport results at low temperature and evolution ofHCandTC. (a,b) MR measured atT=1.5 K (a) and 5 K (b). Each curve is offset by 3% (a) and 1% (b) for clarity. Butterfly-shaped hysteresis confirms the FM order at low temperature. The negative MR is due to local magnetic order induced spin-dependent scattering.TCreaches a minimum at +2 V and increases on both sides, indicating enhanced FM order in bothp- andn-type regime. The increasing temperature reduces theHCand relative change of MR. (c) Summary of theHCandTCat various gate voltages.TCis defined as the temperature whenHCreaches zero within experimental uncertainty. Error bar is due to the discrete temperature points in the measurements. The asymmetry behaviour of theVg-dependentTCsuggests that the hole-doped regime has stronger FM order. MR behaviour of the FM TI film Figure 2a illustrates the H -dependent MR ratio, defined as Figure 2: Magnetotransport results at low temperature and evolution of H C and T C . ( a , b ) MR measured at T =1.5 K ( a ) and 5 K ( b ). Each curve is offset by 3% ( a ) and 1% ( b ) for clarity. Butterfly-shaped hysteresis confirms the FM order at low temperature. The negative MR is due to local magnetic order induced spin-dependent scattering. T C reaches a minimum at +2 V and increases on both sides, indicating enhanced FM order in both p - and n -type regime. The increasing temperature reduces the H C and relative change of MR. ( c ) Summary of the H C and T C at various gate voltages. T C is defined as the temperature when H C reaches zero within experimental uncertainty. Error bar is due to the discrete temperature points in the measurements. The asymmetry behaviour of the V g -dependent T C suggests that the hole-doped regime has stronger FM order. Full size image measured at T =1.5 K under varied gate voltages (the raw ρ xx versus H curves are documented in Supplementary Note 2 ). The butterfly-shaped hysteresis is characteristic of the negative MR in FM metals caused by the spin-dependent scattering of carriers by local magnetic ordering [2] . The peak position corresponds to the coercive field ( H C ), and on either side of H C the reduced scattering of a specific spin orientation leads to negative MR. When V g is reduced to 0 from ±15 V, H C decreases monotonically. The MR behaviour at T =5 K ( Fig. 2b ) is similar, except that the H C value is much smaller (note the change of scale). Figure 2c summarizes the V g and T dependence of H C in a colour contour plot. The general trend is a ‘V’-shaped pattern with apparent asymmetry, where the hole-doped side has stronger FM order. The Curie temperature T C can be estimated from the temperature when H C drops to 0, as shown by the thick blue line. The contour plot clearly demonstrates the enhanced FM order on both sides of the DP, when more carriers are injected into the film by electrical field. The same conclusion can be drawn from the contour plot of gate-tuned anomalous Hall effect shown in Supplementary Fig. 3 . In fact this ‘V’-shaped gate voltage dependence of H C was already present, although totally overlooked, in our previous work on a similar magnetic TI [17] . As shown clearly in Fig. 2a of ref. 17 , H C is smallest around V g =−1.5 V, when E F lies in the magnetic gap at the DP and anomalous Hall effect is quantized. H C increases on either side of the DP (for example, the V g =−55 and 200 V curves apparently have larger H C than the V g =−1.5 V curve), in good agreement with the trend observed here. The MR behaviour at higher temperatures is even more perplexing. 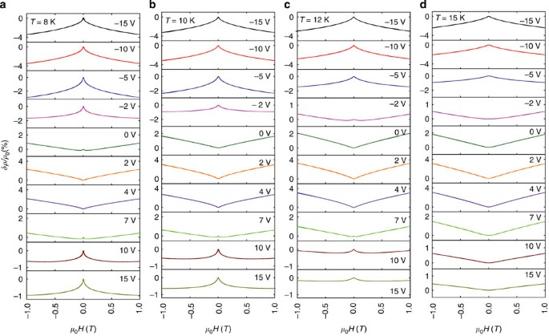Figure 3: Evolution between magnetism-induced negative MR and topology-induced WAL. Gate voltage dependence of MR at various temperatures. AtT=8 K (a) magnetism-induced negative MR at −15 V gradually evolves to the topology-induced WAL behaviour as the gate voltage is swept to +2 V, but with further increase ofVgup to +15 V the MR becomes negative again as that in thep-type regime. Similar trend is observed atT=10 K (b) 12 K (c) and 15 K (d). Figure 3a displays the V g -dependent MR curves measured at T =8 K. The V g =−15 V curve still shows the negative MR similar to that observed at lower temperatures, except that the hysteresis is barely visible due to much reduced H C . With decreasing negative V g to −2 V, the negative MR remains qualitatively the same although the amplitude keeps decreasing. At V g =0 V, the MR is still negative at very weak H , but crossovers to positive for H >0.1 T. At positive V g up to +4 V, the MR exhibits a sharp positive increase with H , but at V g =+7 V the curve returns to the behaviour similar to that at V g =0 V with a negative dip at weak H and a slow positive increase at higher H . With further increase of positive V g up to +15 V, the MR behaviour becomes the same to the regime with large negative V g , showing strongly negative MR. This unusually complex evolution of MR with varied V g is also seen at higher temperatures. The main change with increasing T is in general the positive MR becomes more pronounced. Figure 3: Evolution between magnetism-induced negative MR and topology-induced WAL. Gate voltage dependence of MR at various temperatures. At T =8 K ( a ) magnetism-induced negative MR at −15 V gradually evolves to the topology-induced WAL behaviour as the gate voltage is swept to +2 V, but with further increase of V g up to +15 V the MR becomes negative again as that in the p -type regime. Similar trend is observed at T =10 K ( b ) 12 K ( c ) and 15 K ( d ). 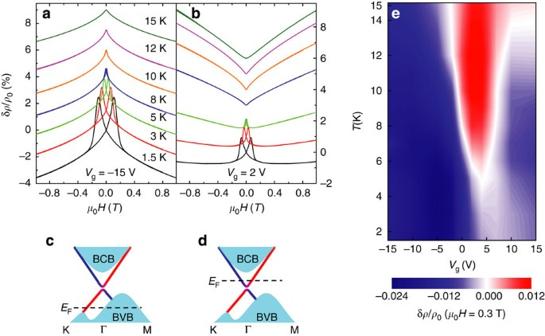Figure 4: Correlation between negative MR and ferromagnetism. (a,b) Temperature dependence of MR at two representative gate voltages. (a)Vg=−15 V. As theEFcuts through the bulk valence band, negative MR is observed over all temperature. Each curve is offset by 1.5% for clarity. (b)Vg=2 V. When theEFis tuned into the bulk gap, WAL begin to take charge the transport and WAL is observed aboveTC. Each curve is offset by 1% for clarity. (c,d) The position ofEFat the two gate voltagesVg=−15 V (c) andVg=+2 V (d). (e) Colour plot of the relative change of MR atμ0H=0.3 T. Negative MR is more pronounced in the regime of highVgand low temperature, which are favourable for the enhancement of ferromagnetism. Full size image Correlation between MR and ferromagnetism Figure 4a,b summarizes the T -dependent MR curves measured at two representative gate voltages. The position of E F corresponding to each V g is shown in the schematic band structure in Fig. 4c,d . It is clear that when E F lies way below the DP ( V g =−15 V) and cuts through the bulk valence band, the negative MR behaviour dominates at all temperatures. In contrast, when E F lies close to the DP ( V g =+2 V) and within the bulk band gap, MR becomes positive for the whole H range for T ≥ T C =8 K, as well as the large H regime for T < T C . Similar T -dependent MR curves measured at other values of V g are shown in Supplementary Fig. 4 . The overall evolution of MR can be directly visualized in Fig. 4e , where a colour scale is used to characterize the relative MR ratio measured at μ 0 H =0.3 T, which is beyond the H C of all curves to avoid complications from hysteresis. Interestingly, there is a close correlation between the MR ratio shown here and the H C plot in Fig. 2e , both showing a ‘V’-shaped pattern centred around V g =+2V. In particular, negative MR is favoured in the regime with stronger ferromagnetism, both in terms of temperature and gate voltage. The same pattern can also be seen in the contour plot of MR taken at other magnetic fields (See Supplementary Note 5 for details). Figure 4: Correlation between negative MR and ferromagnetism. ( a , b ) Temperature dependence of MR at two representative gate voltages. ( a ) V g =−15 V. As the E F cuts through the bulk valence band, negative MR is observed over all temperature. Each curve is offset by 1.5% for clarity. ( b ) V g =2 V. When the E F is tuned into the bulk gap, WAL begin to take charge the transport and WAL is observed above T C . Each curve is offset by 1% for clarity. ( c , d ) The position of E F at the two gate voltages V g =−15 V ( c ) and V g =+2 V ( d ). ( e ) Colour plot of the relative change of MR at μ 0 H =0.3 T. Negative MR is more pronounced in the regime of high V g and low temperature, which are favourable for the enhancement of ferromagnetism. Full size image It is very puzzling why the MR has such a complex evolution with gate voltage. In conventional FM metals or diluted magnetic semiconductors, the amplitude of MR may depend on carrier density [18] but a sign change is rare. Here, we show that in a FM TI film, the sign of MR can change twice as the gate voltage is varied between ±15 V at certain temperature range ( Fig. 3a–c ). Next, we will unravel the mechanism of this peculiar behaviour, which represents a novel transport phenomenon in TIs with spontaneous FM order. At first glance, the results shown in Fig. 3 are reminiscent of the crossover between WAL and weak localization (WL) proposed for magnetically doped TI [19] , but a closer examination of the data suggests otherwise. In pristine TI, spin-momentum locking of the Dirac cone induces a π Berry phase between two time-reversed self-crossing loops [20] . The destructive quantum interference between them leads to WAL, and magnetic field penetrating the loops suppresses the interference and causes a positive MR [11] , [21] , [22] . WAL indicates that the Dirac fermions cannot be localized by nonmagnetic impurities, which is a key aspect of the topological protection [3] , [5] . Magnetism introduced into TI breaks the TRS and opens a gap at the DP [23] , [24] . The Berry phase φ in this case can be expressed as: which depends on the gap size Δ and position of E F (ref. 19 ). When E F lies close to the DP, φ approaches zero, thereby MR should be negative due to WL. However, Fig. 3 shows that MR is positive for E F close to DP and becomes negative for E F at higher energies. This trend is totally opposite to that predicted by the Berry phase picture and indicates that novel physics beyond simple localization must be at work. We gain key insight into this puzzle from the intimate relationship between MR and ferromagnetism. Let’s first focus on the limit of V g =−15 V, which has the strongest FM order. Here, E F cuts through the bulk valence band so that bulk holes make dominant contribution to charge transport ( Fig. 4c ). At low temperatures ( T ≤5 K) the MR is negative with pronounced butterfly-shaped hysteresis, which is the same as that commonly observed in FM metals due to the spin-dependent scattering of charge carriers. With increasing temperature to above T C , the long-range FM order vanishes but strong FM fluctuations make the physics still valid. As shown in Fig. 4a , from 1.5 to 15 K, the MR curves remain qualitatively the same except for the gradual disappearance of H C . The negative MR of the bulk carriers in FM TI thus has little difference from the magnetism-induced negative MR in conventional FM metals, which is not totally unexpected. The irrelevance of the WL picture in this regime is further supported by the unphysical fitting parameters when we use the Hikami–Larkin–Nagaoka formula for localization [23] to simulate the magnetoconductivity curves (see Supplementary Note 6 for details). As E F is moved towards DP by the gate voltage ( V g =+2 V), the charge transport predominantly comes from the surface states because E F lies in the bulk gap ( Fig. 4d ). At T ≥ T C =8 K, there is no long-range FM order; thus, the Dirac cone is gapless. The positive MR in this regime is characteristic of the WAL of surface Dirac fermions, just like that in pristine TI. In this regime, the magnetoconductivity curves can be fitted very well by the Hikami–Larkin–Nagaoka formula with reasonable parameters showing the WAL behaviour ( Supplementary Fig. 6 ). On cooling to below T C , however, the system shows the butterfly-shaped negative MR at weak H . Therefore, even the surface Dirac fermions exhibit rather conventional spin-dependent scattering with local magnetization. As has been shown by recent angle-resolved photoemission spectroscopy measurements, the long-range FM order opens a gap at the DP [24] and leads to a hedgehog spin texture for states outside the magnetic gap [25] . The spins of the Dirac fermions in this regime obtain an out-of-plane component, and will suffer spin-dependent scattering with the local magnetization. Now the massive Dirac fermions behave more like conventional fermions due to the suppression of topological protection by broken TRS. Only at H higher than H C does the MR recover the positive tendency, manifesting the WAL due to residual topological protection. Therefore, the perplexing MR behaviour actually reflects the competition between topology-induced WAL and magnetism-induced negative MR. In the large V g regime where FM order is stronger and bulk conduction prevails, MR is negative in a similar manner to conventional FM metal. In the V g range when E F lies in the bulk gap and surface Dirac fermions are mainly responsible for charge transport, MR is positive due to the WAL effect except for the weak field regime in the FM state. The MR behaviour at intermediate V g can be described as the competition of these two effects ( Supplementary Fig. 3 ). The versatile electrical control of ferromagnetism and MR also allow us to construct novel spintronic and topological magnetoelectric devices using magnetic TIs. For example, the fact that the sign of MR switches twice when V g is changed between ±15 V may be used to achieve novel magnetic readout and signal transmission functions. In certain sense, this is analogous to the famous single electron transistor, which turns on and off again every time one electron is added to the quantum dot by V g (ref. 26 ). The only remaining question is why the FM order is strengthened by increased carrier density ( Fig. 2c ). The origin of magnetism in TI has attracted much recent attention. Available proposals include the bulk van Vleck mechanism [27] and surface Dirac fermion mediated Ruderman–Kittel–Kasuya–Yosida (RKKY) mechanism [28] . The former one is insensitive to the carrier density [15] , whereas in the latter one FM order becomes weaker when E F moves away from the DP [29] . Our gate tuning results provide a new trend that has never been reported before. The enhanced FM order at heavily electron- and hole-doped regime, when the charge transport is dominated by bulk carriers, suggests that the RKKY mechanism involving itinerant bulk carriers is also essential. In fact, it has been shown that in Cr-doped Sb 2 Te 3 , the bulk valence band holes plays an important role in ferromagnetism [13] , but it has yet to be revealed if the bulk conduction-band electrons can do the same thing. Our experimental data shown in Fig. 2c suggest so, although there is an apparent electron-hole asymmetry. This is different from the well-known III–V group diluted magnetic semiconductor, in which only hole-type RKKY is available [30] . A plausible reason is that the TIs have inverted bulk band structure, in which the original bulk conduction/valence bands are hybridized thus share common characteristics. Therefore, bulk electrons can mediate FM order in a similar manner to the bulk band holes, which is unique to the TIs. We note that further theoretical studies with realistic band structure of magnetically doped TI will be needed to confirm this hypothesis. Sample growth and device fabrication The Cr 0.15 (Bi 0.1 Sb 0.9 ) 1.85 Te 3 TI thin film with thickness of five quintuple layers is grown on insulating SrTiO 3 (111) substrate by using molecular beam epitaxy. The film is covered with 10 nm Te capping layer before being taken out of the molecular beam epitaxy chamber. A 50-nm-thick amorphous Al 2 O 3 film deposited by atomic layer deposition is used as the dielectric layer for the top gate. The sample is fabricated into a Hall bar geometry by using photolithography. The length between the longitudinal contacts is 50 μm and width of the sample is 50 μm. Electric contacts are made by mechanically pressing Indium into the film. The 2D Hall resistivity ρ yx and longitudinal resistivity ρ xx are measured by using standard four-probe ac lock-in method with the magnetic field applied perpendicular to the film plane. How to cite this article: Zhang, Z. et al. Electrically tuned magnetic order and magnetoresistance in a topological insulator. Nat. Commun. 5:4915 doi: 10.1038/ncomms5915 (2014).